Hydrotrifluoromethylation and iodotrifluoromethylation of alkenes and alkynes using an inorganic electride as a radical generator The trifluoromethyl (CF 3 ) group is a staple synthon that can alter the physical and chemical properties of organic molecules. Despite recent advances in trifluoromethylation methods, the development of a general synthetic methodology for efficient and selective trifluoromethylation remains an ongoing challenge motivated by a steadily increasing demand from the pharmaceutical, agrochemical and materials science industries. In this article, we describe a simple, efficient and environmentally benign strategy for the hydrotrifluoromethylation of unactivated alkenes and alkynes through a radical-mediated reaction using an inorganic electride, [Ca 2 N] + ·e − , as the electron source. In the transformation, anionic electrons are transferred from [Ca 2 N] + ·e − electrides to the trifluoromethylating reagent CF 3 I to initiate radical-mediated trifluoromethylation. The role of ethanol is pivotal in the transformation, acting as the solvent, an electron-releasing promoter and a hydrogen atom source. In addition, iodotrifluoromethylation of alkynes proceeds selectively upon the control of electride amount. The incorporation of trifluoromethyl groups into organic molecules can markedly alter a myriad of physical and chemical properties of organic compounds because of its strong electron-withdrawing nature and large hydrophobic area [1] , [2] . In particular, trifluoromethylated compounds are characterized by superior metabolic stability, binding selectivity, bioavailability and lipophilicity compared with those of their non-trifluoromethylated analogues, and these characteristics have stimulated the intensive development of new pharmaceutical and agrochemical agents bearing this moiety [3] , [4] , [5] . In general, transition-metal-catalysed cross-coupling reactions (for example, those involving Cu, Pd, Ru or Ir) are regarded as state-of-the-art methods for C–CF 3 bond formation [6] , [7] , [8] , [9] , [10] , [11] , [12] , [13] , [14] , [15] , [16] , [17] , [18] . However, these transition-metal-catalysed reactions pose their own challenges. For example, the presence of potentially toxic transition-metal contaminants in pharmaceuticals is a concern because they may cause adverse effects to human health. In addition, the major procedures in these reactions are somewhat complicated and involve the use of several reagents or additives to achieve high yields of trifluoromethylated products. Therefore, a new approach to trifluoromethylation with a much simpler procedure that maintains high efficiency and selectivity compared with those afforded by transition-metal catalysis is still highly desirable. Recently, inorganic electrides, which are stoichiometric ionic crystals with electrons trapped in cavities acting as anions, have emerged as functional materials in chemistry and materials science [19] , [20] , [21] . The most characteristic feature of electrides—a low work function that originates from the loosely bound anionic electrons to countercations—makes this materials promising electron sources [22] . The recent discovery of the two-dimensional electride dicalcium nitride ([Ca 2 N] + ·e − ), which exhibits a low work function (2.6 eV) and an extremely high electron concentration (~1.37 × 10 22 cm −3 ; ref. 23 ), provides a new opportunity for the broad use of electrides as electron donors in organic reactions under mild conditions. Importantly, electrides can be used in alcohol solvents because an alcohol can act not only as a ligand to stabilize the calcium cations but also as a medium for electron transfer. In addition, alcohols can be used as hydrogen atom sources. By taking advantage of the versatile utility of alcohols, we developed a simple and convenient procedure for hydrotrifluoromethylation method by the addition of electrides in alcohols ( Fig. 1b ). 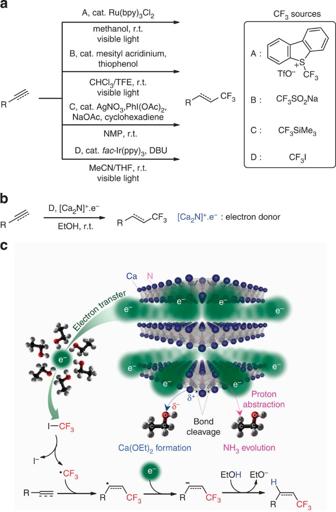Figure 1: Hydrotrifluoromethylation of alkenes and alkynes. (a) Previous reports of hydrotrifluoromethylation. (b) Hydrotrifluoromethylation using [Ca2N]+·e−as the electron donor. (c) Working model of the electride and the roles of EtOH. THF, tetrahydrofuran; TFE: 2,2,2-trifluoroethanol; DBU, 1,8-diazabicyclo[5.4.0]undec-7-ene; NMP,N-methyl-2-pyrrolidone; cat., catalyst; r.t., room temperature. Figure 1: Hydrotrifluoromethylation of alkenes and alkynes. ( a ) Previous reports of hydrotrifluoromethylation. ( b ) Hydrotrifluoromethylation using [Ca 2 N] + ·e − as the electron donor. ( c ) Working model of the electride and the roles of EtOH. THF, tetrahydrofuran; TFE: 2,2,2-trifluoroethanol; DBU, 1,8-diazabicyclo[5.4.0]undec-7-ene; NMP, N -methyl-2-pyrrolidone; cat., catalyst; r.t., room temperature. Full size image The trifluoromethylation of alkenes and alkynes is relatively underdeveloped compared with the trifluoromethylation of arenes and heteroarenes [24] , [25] , [26] , [27] , [28] , [29] , [30] , [31] , [32] , [33] . In particular, the literature contains only a few reports of the hydrotrifluoromethylation of alkenes and alkynes [34] , [35] , [36] , [37] . Here, we report an environmentally benign, efficient and simple method for a radical-initiated hydrotrifluoromethylation reaction with alkenes and alkynes using the inorganic electride [Ca 2 N] + ·e − as an electron donor. This protocol may provide an attractive complement to transition-metal catalysis in terms of the minimization of waste from CF 3 sources, the reduced use of additives and the avoidance of costs associated with the use of precious-metal catalysts. In the presence of an alcohol solvent, loosely bound electrons are easily released from the open-layer-structured [Ca 2 N] + ·e − to form NH 3 and Ca(OEt) 2 , which are easily removed by an aqueous workup. Optimization for hydrotrifluoromethylation of alkenes The investigation was initiated by using styrene 1a as a model substrate and CF 3 I [38] with [Ca 2 N] + ·e − as the electron source in alcohol solvents, and the effects of several solvents, additives and concentrations were systematically examined. As revealed in Table 1 , the solvents strongly influenced the reaction. The use of either MeOH or EtOH delivered the expected product in low-to-moderate yield (entries 1 and 2). The [Ca 2 N] + ·e − likely reacted vigorously with alcohol and thus released electrons too quickly to match the electron transfer rate to CF 3 I. The use of an aprotic co-solvent (for example, CH 2 Cl 2 or MeCN) tended to slow down the activation of the electride, thereby markedly enhancing the reaction yields. The highest activity of the electride was observed when a mixture of ethanol and MeCN in a 1:1 ratio was used (entry 5). Increased solubility of CF 3 I in MeCN may also contribute to the increased reactivity. However, it should be noted that the reaction did not proceed in the absence of an alcohol solvent, provoking the further clarification of solvent effect on electride activity. With respect to the styrene concentration, a 0.1-M mixture was optimal (entries 5, 8 and 9). The product yield was significantly decreased when the equivalents of electride were decreased ( Table 1 , entry 10). The addition of an additional hydrogen atom source, HCO 2 H, deactivated the transformation (entry 12). Table 1 Optimization studies for the hydrotrifluoromethylation of styrene * . Full size table Solvent effect To ensure the direct reaction of electrides with alcoholic solvents and verify the vital role of a solvent system on the electride activity, the decomposition of structure along with the consumption of electrons in [Ca 2 N] + ·e − were examined after reacting with only solvents such as a pure ethanol and mixture of ethanol and MeCN in a 1:1 ratio. The reaction time dependences of X-ray diffraction (XRD) pattern and iodometric titration clearly showed that the electrides directly reacted with ethanol and the rates of structure decomposition and electron consumption are highly vigorous in a pure ethanol solvent ( Fig. 2a ). Meanwhile, it is noteworthy that the decomposition was suppressed by using co-solvent system adding acetonitrile to ethanol ( Fig. 2b ). This indicates that the mixed solvent system provides more favourable condition for the present hydrotrifluoromethylation than a pure ethanol solvent by contributing to the slow decomposition of [Ca 2 N] + ·e − structure and steady generation of electrons ( Fig. 2b and Supplementary Table 1 ). Details of XRD analysis and iodometric titrations are described in the Supplementary Methods . 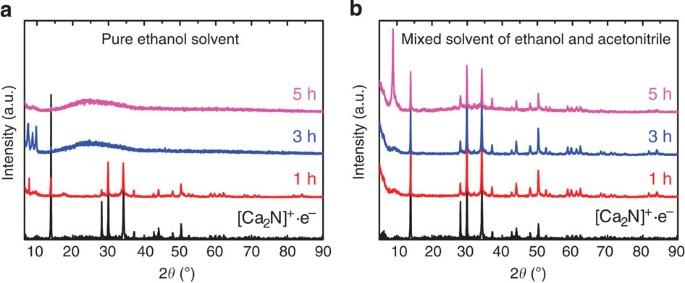Figure 2: XRD analysis of [Ca2N]+·e−. XRD patterns of dicalcium nitride [Ca2N]+·e−powders (black line) and resultant powder products after reacting with (a) pure ethanol (5 ml) and (b) mixture (5 ml) of ethanol and acetonitrile in a 1:1 ratio. The red, blue and pink colour represents the reaction time of 1, 3 and 5 h, respectively. All measurements are performed under inert Ar atmosphere. The sharp and broad peaks appeared at 8° and 23° are attributed to the formation of Ca(OEt)2and gel-like products, respectively. The formation of gel-like products indicates that the electrides directly reacts with ethanol in a short time, decomposing the structure and consuming the electrons. Figure 2: XRD analysis of [Ca 2 N] + ·e − . XRD patterns of dicalcium nitride [Ca 2 N] + ·e − powders (black line) and resultant powder products after reacting with ( a ) pure ethanol (5 ml) and ( b ) mixture (5 ml) of ethanol and acetonitrile in a 1:1 ratio. The red, blue and pink colour represents the reaction time of 1, 3 and 5 h, respectively. All measurements are performed under inert Ar atmosphere. The sharp and broad peaks appeared at 8° and 23° are attributed to the formation of Ca(OEt) 2 and gel-like products, respectively. The formation of gel-like products indicates that the electrides directly reacts with ethanol in a short time, decomposing the structure and consuming the electrons. Full size image Substrate scope for hydrotrifluoromethylation of alkenes A variety of styrene derivatives were explored under optimized conditions ( Table 2 ). In a short reaction time (0.5–2 h), both electron-rich and electron-poor styrene derivatives underwent hydrotrifluoromethylations in good-to-excellent yields. Notably, the desired hydrotrifluoromethylated products were selectively formed, despite being hampered by side reactions, such as aryl-trifluoromethylation and dehalogenation from the aromatic moiety. Trifluoromethylation did not proceed on the aromatic moiety of styrene derivatives under the optimized conditions to selectively give hydrotrifluoromethylated products on the alkene moiety ( Fig. 3 (1) and (2); ref. 13 ). These observations indicate that alkenes are better radical acceptors than aromatics, and that the benzylic radical is more stable than the aryl radical. Another possible competitive pathway is the dehalogenation of halogenated styrene substrates because aryl halides can also accept an electron to form an aryl radical, which further undergoes hydrogen abstraction from EtOH ( Fig. 3 (3); refs 39 , 40 ). While the reaction of 4-bromostyrene 1e in the absence of CF 3 I provided debromonated product 1e′ ( Fig. 3 (4)), no detectable amounts of debromonated products, 1e′ or 2e′ , were observed in the presence of CF 3 I (entry 5 in Table 2 and Fig. 3 (5)). The results strongly indicate that hydrotrifluoromethylation is much more kinetically favourable than dehalogenation under the given conditions ( Table 2 , entries 3–5). 1,1-Disubstituted alkenes such as α-methylstyrene also gave the hydrotrifluoromethylated product ( Table 2 , entry 6). Table 2 Hydrotrifluoromethylation of aromatic alkenes * . 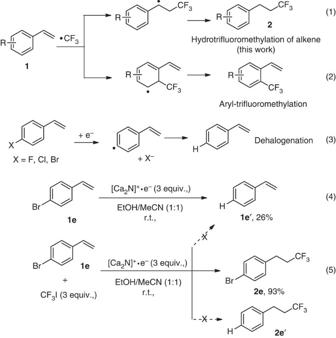Figure 3: Suppression of possible side reactions. Selective hydrotrifluoromethylation on the alkene moiety over the aromatic moiety [(1) and (2)] and suppression of dehalogenation [(3), (4), and (5)]. Full size table Figure 3: Suppression of possible side reactions. Selective hydrotrifluoromethylation on the alkene moiety over the aromatic moiety [(1) and (2)] and suppression of dehalogenation [(3), (4), and (5)]. Full size image Furthermore, perfluoro-tagged long alkyl groups were also installed on styrene derivatives 1a and 1e in good yields using heptafluoropropyl iodide and non afluorobutyl iodide, which can be attributed to a similar reactivity between C n F 2n+1 I (where n =3 and 4) and CF 3 I ( Fig. 4 ). 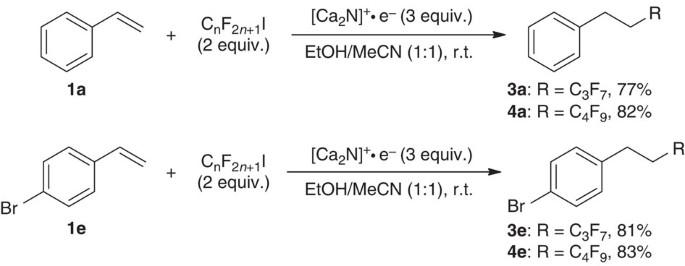Figure 4: Hydroheptafluoroalkylation and hydrononafluoroalkylation of alkenes. Aromatic alkenes are perfluoroalkylated with C3F7I and C4F9I. Figure 4: Hydroheptafluoroalkylation and hydrononafluoroalkylation of alkenes. Aromatic alkenes are perfluoroalkylated with C 3 F 7 I and C 4 F 9 I. Full size image Substrate scope for hydrotrifluoromethylation of alkynes Next, hydrotrifluoromethylation reactions with alkynes were investigated ( Table 3 ). The reactivity of phenylacetylene derivatives for hydrotrifluoromethylation was similar to that of styrene derivatives (entries 1–5). Hydrotrifluoromethylation of both electron-rich and electron-poor phenylacetylene derivatives with CF 3 I smoothly proceeded in EtOH/MeCN (v/v=1:1, 0.1 M) when the electride [Ca 2 N] + ·e − was used to produce an E / Z mixture of alkenyl–CF 3 compounds in good-to-excellent yields. Alkynes with a heteroaromatic substituent, such as 5e , also underwent selective hydrotrifluoromethylation on the alkyne moiety (entry 5). In cases of aliphatic alkynes ( 5f–5j ), 4 equiv. of [Ca 2 N] + ·e − was required to obtain good yields of the desired hydrotrifluoromethylated products (entries 6–10). The reaction conditions allowed hydrotrifluoromethylation of alkynes containing unprotected alcohol ( 5i ) and amine ( 5j ). Collectively, the resulting alkenyl–CF 3 products ( 6a – 6j ) were considerably less reactive towards further possible double hydrotrifluoromethylation, thereby showing high selectivity of the mono-hydrotrifluoromethylation of alkynes. Table 3 Hydrotrifluoromethylation of alkynes * . Full size table Iodotrifluoromethylation of aliphatic alkynes It is noteworthy that the iodotrifluoromethylated product can also be obtained using <2 equiv. of [Ca 2 N] + ·e − in the reactions of aliphatic alkynes ( Table 4 ). The use of 1.5 equiv. of [Ca 2 N] + ·e − led to the selective iodotrifluoromethylation of alkynes with an excellent E/Z selectivities. This approach provides an attractive platform for green chemistry since carbon–carbon and carbon–halide bonds are simultaneously formed in a straightforward and atom economical fashion. The resulting alkenyl iodide products are valuable CF 3 -building blocks since they can easily be converted by various cross-coupling reactions into CF 3 -containing tri-substituted alkenes, commonly found as a structural motif in pharmaceuticals and agrochemicals. Table 4 Iodotrifluoromethylation of aliphatic alkynes * . Full size table Mechanistic studies To propose a mechanism for the hydrotrifluoromethylating process using [Ca 2 N] + ·e − , several experiments were further conducted. First, the reaction of 1a was conducted in the presence of various radical scavengers, such as TEMPO, galvinoxyl, or 1,4-dinitrobenzene, under optimized conditions ( Supplementary Table 2 ). These controlled experiments showed that the reaction was suppressed, indicating that a radical species is involved via a single-electron transfer (SET) mechanism in the transformation. To ascertain mechanistic insight into the source of hydrogen, isotopic labeling experiment was conducted with ethanol- d 1 (C 2 H 5 OD). Hydroperfluoroalkyations of either styrene 1a or phenylacetylene 5a with 3 equiv. of [Ca 2 N] + ·e − were performed in a 1:1 mixture of EtOD and acetonitrile ( Fig. 5 ). The deuterated products ( 2a′ , 4a′ and 6a′ ) were exclusively formed from the reactions, clearly confirming that the hydrogen of the –OH group on the ethanol is the actual source of hydrogen in this process. Namely, no hydrogen abstraction from α-C–H bond of ethanol occurred [34] , [35] . 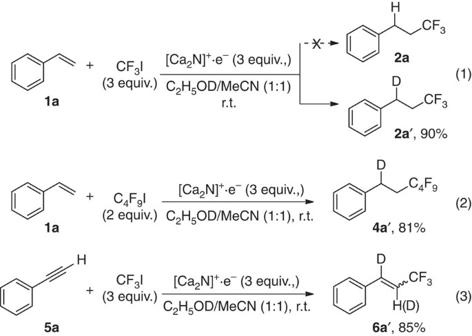Figure 5: Hydroperfluoroalkylation in EtOD/MeCN (v/v=1:1). The use of EtOD generates the deuterated products confirming that –OH group of ethanol is the hydrogen atom source in the hydroperfluoroalkylation process. Figure 5: Hydroperfluoroalkylation in EtOD/MeCN (v/v=1:1). The use of EtOD generates the deuterated products confirming that –OH group of ethanol is the hydrogen atom source in the hydroperfluoroalkylation process. Full size image Proposed mechanism Based on these results, we propose a plausible mechanism for this simple hydrotrifluoromethylation in Fig. 6 . An SET from [Ca 2 N] + ·e − to CF 3 I results in the simultaneous formation of a carbon-centered CF 3 radical and an iodide anion. The addition of electron-deficient CF 3 radical to an alkene or alkyne generates alkyl or vinyl radicals, respectively. In this process, ethanol is used as an electride activator and also as a hydrogen donor, eliminating the need for an additional hydrogen source. Although we cannot rule out the direct hydrogen abstraction of an alkyl/vinyl radical from ethanol (pathway (a) in Fig. 6 ) [34] , it is highly likely that the hydrotrifluoromethylated product is formed through alkyl or vinyl carbanion formation by the second SET from [Ca 2 N] + ·e − to the radical and its protonation (pathway (b)) based on the results conducted in EtOD shown in Fig. 5 . Notably, the alkyl/vinyl radical, when R is aliphatic, is less reactive towards the second SET from [Ca 2 N] + ·e − , and thus the process of aliphatic substrates requires more amount of electrides (4 equiv.). The use of <2 equiv. [Ca 2 N] + ·e − leads to competitive pathway, iodine abstraction of the alkyl/vinyl radical from CF 3 I to generate an iodotrifluoromethylated product and a CF 3 radical (pathway (c)). Specifically, reactions of aliphatic alkenes produced a mixture of iodotrifluoromethylated and hydrotrifluoromethylated compounds, whereas those of aliphatic alkynes provided trifluoromethylated alkenyl iodide as the exclusive product with 1.5 equiv. [Ca 2 N] + ·e − , as shown in Table 4 . 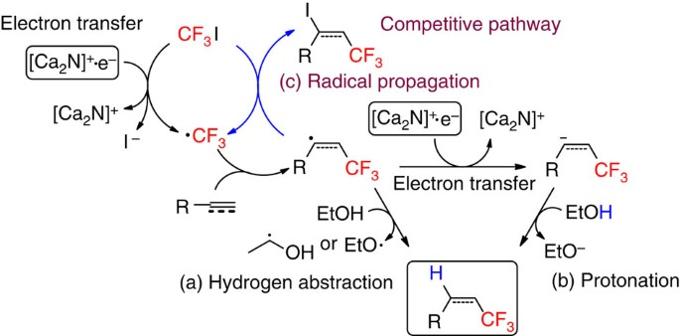Figure 6: Proposed mechanism of hydrotrifluoromethylation or iodotrifluoromethylation of alkenes and alkynes. Formation of hydrotrifluoromethylated product from alkyl/vinyl radical intermediates by (a) direct hydrogen abstraction or (b) further reduction followed by protonation, and generation of iodotrifluoromethylated product by radical propagation (3) with CF3I. Figure 6: Proposed mechanism of hydrotrifluoromethylation or iodotrifluoromethylation of alkenes and alkynes. Formation of hydrotrifluoromethylated product from alkyl/vinyl radical intermediates by (a) direct hydrogen abstraction or (b) further reduction followed by protonation, and generation of iodotrifluoromethylated product by radical propagation (3) with CF 3 I. Full size image We have demonstrated a simple, efficient and convenient method for the hydrotrifluoromethylation of unactivated alkenes and alkynes with CF 3 I using an inorganic electride as an electron source via an SET pathway. The ability to use ethanol as a hydrogen atom source obviated the use of additives, and thus this reaction process requires only electride [Ca 2 N] + ·e − in ethanol/MeCN. In addition, the heterogeneous reaction conditions excluded an intricate or laborious procedure for product isolation, and even by-products of the process are environmentally benign and easily separable from the crude product mixture. We present our protocol as one of the most practical trifluoromethylation reactions and a possible milestone for the application of electrides in synthetic organic chemistry. Synthesis of [Ca 2 N] + ·e − Stoichiometric polycrystalline [Ca 2 N] + ·e − was synthesized by the solid-state reaction of calcium nitride (Ca 3 N 2 ) powder and calcium metal. Mixtures of Ca 3 N 2 powder and calcium chips at a molar ratio of 1:1 were pressed into a pellet under 30 MPa of pressure. The pellet was covered with molybdenum foil and annealed at 800 °C for 48 h under vacuum (~10 −3 Pa). The sample was subsequently quenched in water. To improve the homogeneity of [Ca 2 N] + ·e − , the synthesized sample was ground into a powder in an agate mortar in a nitrogen-filled glove box and re-annealed under the same conditions. General experimental procedure In a nitrogen-filled glove box, an oven-dried re-sealable test tube equipped with a magnetic stir bar was charged with [Ca 2 N] + ·e − (141 mg, 1.5 mmol). The tube was then sealed with a screw cap and removed from the glove box. A premixed solution of an alkene or an alkyne (0.5 mmol) in EtOH/MeCN (2.5:2.5 ml) was transferred to the tube containing the electride. CF 3 I (1.5 mmol) was then bubbled into the reaction mixture using a gas-tight syringe. The reaction was allowed to proceed for 0.5–2 h at room temperature. The reaction mixture was then diluted with EtOAc or dichloromethane (when the product was volatile) and washed with water. The organic layers were dried over MgSO 4 , concentrated in vacuo and purified by flash column chromatography to give the product. The details of hydrotrifluoromethylation, iodotrifluoromethylation, hydroheptafluoroalkylation and hydrononafluoroalkylation are described in the Supplementary Methods . For nuclear magnetic resonance analysis of the compounds in this article, see the Supplementary Methods and Supplementary Figs 1–46 . How to cite this article : Choi, S. et al . Hydrotrifluoromethylation and iodotrifluoromethylation of alkenes and alkynes using an inorganic electride as a radical generator. Nat. Commun. 5:4881 doi: 10.1038/ncomms5881 (2014).